An MTCH2 pathway repressing mitochondria metabolism regulates haematopoietic stem cell fate The metabolic state of stem cells is emerging as an important determinant of their fate. In the bone marrow, haematopoietic stem cell (HSC) entry into cycle, triggered by an increase in intracellular reactive oxygen species (ROS), corresponds to a critical metabolic switch from glycolysis to mitochondrial oxidative phosphorylation (OXPHOS). Here we show that loss of mitochondrial carrier homologue 2 (MTCH2) increases mitochondrial OXPHOS, triggering HSC and progenitor entry into cycle. Elevated OXPHOS is accompanied by an increase in mitochondrial size, increase in ATP and ROS levels, and protection from irradiation-induced apoptosis. In contrast, a phosphorylation-deficient mutant of BID, MTCH2’s ligand, induces a similar increase in OXPHOS, but with higher ROS and reduced ATP levels, and is associated with hypersensitivity to irradiation. Thus, our results demonstrate that MTCH2 is a negative regulator of mitochondrial OXPHOS downstream of BID, indispensible in maintaining HSC homeostasis. Cellular metabolism plays a critical role in determining the fate of stem cells [1] , [2] , [3] . Haematopoietic stem cells (HSCs) are mostly retained in a quiescent non-motile state in their bone marrow niches and shift to a migratory cycling and differentiating state, replenishing the blood with mature leukocytes and red blood cells on demand [4] , [5] . It is well established that ROS drives HSC entry into cycle, and more recently it has been demonstrated that the transition from stem to progenitor cell corresponds to a metabolic switch from glycolysis to mitochondrial oxidative phosphorylation (OXPHOS) [6] , [7] , [8] , [9] , [10] , [11] . Previously, the ataxia–telangiectasia mutated (ATM) kinase was shown to play an important role in regulating the self-renewal and quiescence of HSCs by regulating ROS levels [12] , [13] . More recently we demonstrated that the BH3-interacting domain death agonist (BID) protein acts as a downstream ATM-effector in this pathway and regulates the quiescence of HSCs by balancing ROS levels produced by mitochondria [14] . In our previous study we demonstrated that BID AA HSCs (expressing the non-phosphorylatable BID protein) escape from quiescence. However, the exact mechanism by which BID regulates mitochondrial ROS and its relation to the switch to mitochondrial OXPHOS described in the transition from stem to progenitor cell remained unknown [15] . To address this issue, we shifted our focus to mitochondrial carrier homologue 2 (MTCH2), BID’s receptor-like protein in the mitochondria that plays a critical role in Fas-induced liver apoptosis [16] . Interestingly, many recent genome-wide association studies associate MTCH2 with metabolic disorders including diabetes and obesity, suggesting that MTCH2 also plays a role in metabolism [17] , [18] , [19] . Knockout of mtch2 gene in embryonic stem cells hinders the recruitment of BID to mitochondria [16] , therefore, we hypothesized that MTCH2 serves as a critical regulator of HSC mitochondrial function downstream of ATM and BID. In the present study we demonstrate that loss of MTCH2 primes mitochondrial OXPHOS and drives haematopoietic stem and progenitor cells (HSPCs) into cycle leading to stem cell exhaustion. Similar findings were obtained with our previously described BID AA mice [14] , indicating that MTCH2 is an essential regulator of haematopoietic homeostasis downstream of ATM and BID. Loss of MTCH2 impairs HSC homeostasis To determine whether MTCH2 is critical for maintenance of HSPCs, we generated a genetic mouse model where MTCH2 deletion is driven by the Vav1-Cre allele [20] ( MTCH2 F/F Vav1-cre + ), resulting in haematopoietic-specific knockout of MTCH2 ( Fig. 1a ). Upon MTCH2 deletion, we observed a reduction in the frequency of phenotypic HSCs in the bone marrow (CD150 + CD48 − CD41 − Lin − Sca-1 + c-Kit + ; Fig. 1b ) and apparent increase in restricted progenitor populations (CD150 − CD48 − CD41 − and CD150 − CD48 + CD41 − Lin − Sca-1 + c-Kit + ; Fig. 1c ), indicating perturbed HSC homeostasis in MTCH2 F/F Vav1-cre + mice. Interestingly, however, there was no change in steady-state leukocytes in the blood ( Supplementary Fig. 1 ). Analysing the cell cycle status of MTCH2 F/F Vav1-cre + HSCs and progenitor populations, we observed a reduction in quiescent HSCs ( Fig. 1d ), which was accompanied by increased proliferation of HSCs, HSPCs (Lin − Sca-1 + c-Kit + ; LSK) and committed progenitors (Lin − Sca-1 − c-Kit + ; LK; Fig. 1e ). The observed HSC exhaustion in MTCH2 F/F Vav1-cre + mice resulted in reduced colony-forming capacity ( Fig. 1f ), a competitive disadvantage in bone marrow repopulation ( Fig. 1g ) and increased mobilization to peripheral blood ( Fig. 1h ). These results identify MTCH2 as a novel regulator of HSPC homeostasis in the ATM–BID pathway. 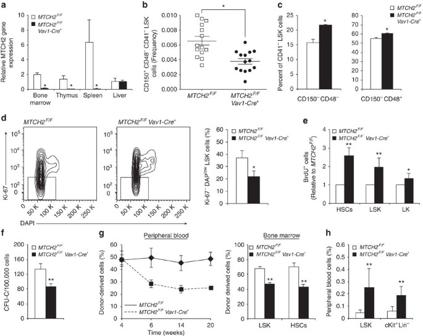Figure 1: Loss of MTCH2 impairs HSC homeostasis. (a) MTCH2-deletion driven byVav1-Creresults in haematopoietic-specificMTCH2knockout. Relative MTCH2 gene expression was evaluated in freshly isolated cells from the indicated tissues by quantitative real-time PCR. Results are presented as mean relative quantity±s.d. (Unpairedt-test, *P≤0.05,n=4). (b) Reduced HSC bone marrow frequency on MTCH2 deletion. Mice were killed and their total bone marrow cells were evaluated by flow cytometry for the size of the indicated populations. Results are presented as mean per cent±s.d. (Unpairedt-test, *P≤0.05,n=14). (c) MTCH2 deletion increases restricted-progenitor levels in the bone marrow. Mice were killed and their total bone marrow cells were evaluated by flow cytometry for the size of the indicated populations. Results are presented as mean per cent±s.d. (Unpairedt-test, *P≤0.05,n=4). (d) MTCH2-deficient HSCs are less quiescent. Quiescent HSCs were evaluated by staining freshly isolated bone marrow cells with anti-Ki-67 antibody coupled with DAPI staining for total DNA. Results are presented as mean±s.d. (Unpairedt-test, *P<0.05,n=4). (e) Enhanced proliferation in MTCH2-deficient HSCs and committed progenitors. Mice were administered BrdU and the levels of incorporation in the indicated populations was evaluated by flow cytometry. Results are presented as means±s.d. (Unpairedt-test, *P≤0.05; **P≤0.005,n=4). (f) MTCH2-deficient bone marrow cells show reduced colony formation ability. Mice were killed and bone marrow mono-nuclei cells were plated and grown as described in the Methods. Results are presented as means±s.d. (Unpairedt-test, **P≤0.005,n=3). (g) MTCH2-deficient cells show competitive disadvantage in bone marrow repopulation. Total bone marrow cells were transplanted at a 1:1 ratio into lethally irradiated hosts and peripheral blood engraftment (left) and bone marrow engraftment (right) were determined by flow cytometry. Results are presented as means±s.d. of donor-derived cells (Unpairedt-test, **P≤0.005,n=5). (h) MTCH2-deficient HSPCs show increased mobilization to peripheral blood. Results are presented as mean±s.d. (Unpairedt-test, **P≤0.005,n=8). Figure 1: Loss of MTCH2 impairs HSC homeostasis. ( a ) MTCH2-deletion driven by Vav1-Cre results in haematopoietic-specific MTCH2 knockout. Relative MTCH2 gene expression was evaluated in freshly isolated cells from the indicated tissues by quantitative real-time PCR. Results are presented as mean relative quantity±s.d. (Unpaired t -test, * P≤ 0.05, n =4). ( b ) Reduced HSC bone marrow frequency on MTCH2 deletion. Mice were killed and their total bone marrow cells were evaluated by flow cytometry for the size of the indicated populations. Results are presented as mean per cent±s.d. (Unpaired t -test, * P≤ 0.05, n =14). ( c ) MTCH2 deletion increases restricted-progenitor levels in the bone marrow. Mice were killed and their total bone marrow cells were evaluated by flow cytometry for the size of the indicated populations. Results are presented as mean per cent±s.d. (Unpaired t -test, * P≤ 0.05, n =4). ( d ) MTCH2-deficient HSCs are less quiescent. Quiescent HSCs were evaluated by staining freshly isolated bone marrow cells with anti-Ki-67 antibody coupled with DAPI staining for total DNA. Results are presented as mean±s.d. (Unpaired t -test, * P< 0.05, n =4). ( e ) Enhanced proliferation in MTCH2-deficient HSCs and committed progenitors. Mice were administered BrdU and the levels of incorporation in the indicated populations was evaluated by flow cytometry. Results are presented as means±s.d. (Unpaired t -test, * P≤ 0.05; ** P≤ 0.005, n =4). ( f ) MTCH2-deficient bone marrow cells show reduced colony formation ability. Mice were killed and bone marrow mono-nuclei cells were plated and grown as described in the Methods. Results are presented as means±s.d. (Unpaired t -test, ** P≤ 0.005, n =3). ( g ) MTCH2-deficient cells show competitive disadvantage in bone marrow repopulation. Total bone marrow cells were transplanted at a 1:1 ratio into lethally irradiated hosts and peripheral blood engraftment (left) and bone marrow engraftment (right) were determined by flow cytometry. Results are presented as means±s.d. of donor-derived cells (Unpaired t -test, ** P≤ 0.005, n =5). ( h ) MTCH2-deficient HSPCs show increased mobilization to peripheral blood. Results are presented as mean±s.d. (Unpaired t -test, ** P≤ 0.005, n =8). Full size image Loss of MTCH2 primes mitochondrial OXPHOS To evaluate the effect of MTCH2 knockout on mitochondrial function in HSPCs we initially measured cellular respiration in c-Kit + progenitor-enriched bone marrow cells and revealed an increase in both basal and maximal oxygen consumption of MTCH2 F/F Vav1-cre + progenitors ( Fig. 2a , left and middle panels). Importantly, the MTCH2 knockout enriched progenitors also possess substantial mitochondrial spare respiratory capacity (SRC; Fig. 2a , right panel), which is the extra capacity available in cells to produce energy in response to increased stress and as such is associated with cellular survival [21] . Similar observations have been recently reported, where a deficiency in the glycolytic enzyme lactate dehydrogenase A (LDHA) induces HSC differentiation and is accompanied by an increase in mitochondrial OXPHOS and SRC in HSPCs [22] . 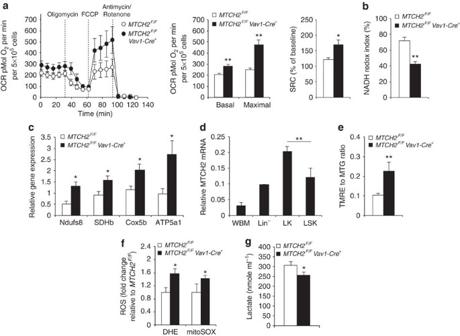Figure 2: Loss of MTCH2 primes mitochondrial OXPHOS. (a) Increased mitochondrial respiration in MTCH2-deficient progenitors. Oxygen consumption rates (OCR) were measured in CD117+enriched progenitors using the Seahorse XF24 analyzer. Basal OCR, Maximal OCR, and Spare Respiratory Capacity (SRC; average results shown in left panel) are shown on the middle and right panels. A representative experiment of four is shown. Results are presented as mean±s.d. (Unpairedt-test, **P≤0.005, *P≤0.05,n=8). (b) Reduced NADH redox in MTCH2-deficient HSPCs. NADH redox index was calculated as described in the Methods. Results are presented as mean per cent±s.d. (Unpairedt-test, **P≤0.005,n=4). (c) Increased expression of nuclear-encoded subunits of the mitochondrial respiratory complexes in MTCH2-deficient progenitors. Results are presented as mean relative quantity±s.d. (Unpairedt-test, *P≤0.05,n=4). (d) Increased MTCH2 expression in LK as compared to LSK cells. LK population (Lin−Sca-1−c-Kit+) and LSK (Lin−Sca-1+c-Kit+) populations were sorted and MTCH2 mRNA levels were evaluated relative to β-actin mRNA level. Results are presented as mean relative quantity±s.d. (Unpairedt-test, **P≤0.005,n=5). (e) Increased mitochondrial membrane potential in MTCH2-deficient HSCs. Results are presented as means±s.d. (Unpairedt-test, **P≤0.005,n=4). (f) Moderate increase in ROS levels in MTCH2-deficient HSCs. Levels of cellular ROS (measured using Dihydroethidium; DHE) and mitochondrial ROS (measured using mitoSOX) are presented. Results are presented as mean±s.d. (Unpairedt-test, *P≤0.05,n=4). (g) Decreased lactate production by MTCH2-deficient CD117+enriched progenitors. Lactate production was assessed as described in the Methods. Results are presented as mean±s.d. (Unpairedt-test, *P≤0.05,n=4). Figure 2: Loss of MTCH2 primes mitochondrial OXPHOS. ( a ) Increased mitochondrial respiration in MTCH2-deficient progenitors. Oxygen consumption rates (OCR) were measured in CD117 + enriched progenitors using the Seahorse XF24 analyzer. Basal OCR, Maximal OCR, and Spare Respiratory Capacity (SRC; average results shown in left panel) are shown on the middle and right panels. A representative experiment of four is shown. Results are presented as mean±s.d. (Unpaired t -test, ** P≤ 0.005, * P≤ 0.05, n =8). ( b ) Reduced NADH redox in MTCH2-deficient HSPCs. NADH redox index was calculated as described in the Methods. Results are presented as mean per cent±s.d. (Unpaired t -test, ** P≤ 0.005, n =4). ( c ) Increased expression of nuclear-encoded subunits of the mitochondrial respiratory complexes in MTCH2-deficient progenitors. Results are presented as mean relative quantity±s.d. (Unpaired t -test, * P≤ 0.05, n =4). ( d ) Increased MTCH2 expression in LK as compared to LSK cells. LK population (Lin − Sca-1 − c-Kit + ) and LSK (Lin − Sca-1 + c-Kit + ) populations were sorted and MTCH2 mRNA levels were evaluated relative to β-actin mRNA level. Results are presented as mean relative quantity±s.d. (Unpaired t -test, ** P≤ 0.005, n =5). ( e ) Increased mitochondrial membrane potential in MTCH2-deficient HSCs. Results are presented as means±s.d. (Unpaired t -test, ** P≤ 0.005, n =4). ( f ) Moderate increase in ROS levels in MTCH2-deficient HSCs. Levels of cellular ROS (measured using Dihydroethidium; DHE) and mitochondrial ROS (measured using mitoSOX) are presented. Results are presented as mean±s.d. (Unpaired t -test, * P≤ 0.05, n =4). ( g ) Decreased lactate production by MTCH2-deficient CD117 + enriched progenitors. Lactate production was assessed as described in the Methods. Results are presented as mean±s.d. (Unpaired t -test, * P≤ 0.05, n =4). Full size image To determine whether the increased respiration observed in the MTCH2-deficient enriched progenitor population correlated with increased respiration in more enriched stem and progenitor cells, we determined mitochondrial NADH levels and redox state in HSPCs (LSK cells), as previously described [23] . As expected, we observed decreased NADH redox due to accelerated electron consumption ( Fig. 2b ) and an expected increase in mitochondrial NADH content ( Supplementary Fig. 2 ), correlating with the enhanced mitochondrial respiratory capacity. Further evaluation of mitochondrial parameters in MTCH2-deleted mice showed an increase in the expression of nuclear-encoded subunits of the respiratory complexes in progenitor-enriched population ( Fig. 2c ). Interestingly, this increase in the expression of respiratory complex subunits was not observed in the LSK cells (not shown), perhaps due to the fact that MTCH2 shows an approximately twofold higher expression level in restricted progenitors (LK population) as compared with HSPCs (LSK population; Fig. 2d ). In addition, MTCH2 knockout increased the mitochondria membrane potential (ΔΨm; Fig. 2e ), and mildly increased both cellular and mitochondrial ROS levels in HSCs ( Fig. 2f ). Interestingly, and as would be expected, the increase in respiration/mitochondrial function was accompanied by a decrease in lactate production in enriched progenitor cells ( Fig. 2g ), indicative of decreased glycolysis. These results identify MTCH2 as a critical suppressor of mitochondrial OXPHOS in HSPCs, and suggest that this suppressive activity is required to prevent excessive differentiation of haematopoietic progenitors leading to HSC exhaustion. Loss of MTCH2 increases mitochondrial size/volume To assess whether the mitochondrial functional changes described above in the MTCH2 F/F Vav1-cre + progenitors were accompanied by changes in mitochondrial structure, we conducted electron microscopy analyses of enriched progenitors. Notably, these analyses revealed that mitochondria of MTCH2 F/F Vav1-cre + progenitors were significantly enlarged ( Fig. 3a , left and middle panels). Interestingly, there was no significant change in the number of mitochondria per cell ( Fig. 3a , right panel), which is consistent with the flow cytometric studies showing no change in mitochondria mass ( Supplementary Fig. 3 ). To obtain a more quantitative analysis of this phenotype, we prepared progenitor-enriched cells by magnetic cell sorting, followed by staining the mitochondria with Mitotracker Red (MitoRed). We then quantified the three-dimensional (3D) volume of mitochondria by computerized segmentation ( Fig. 3b , left and middle panels). We found that the MTCH2 F/F Vav1-cre + cells show an increase in mitochondrial volume as compared with the control MTCH2 F/F cells ( Fig. 3b , right panel). To assess whether loss of MTCH2 in a more stem and progenitor-enriched population also results in an increase in mitochondrial volume, enriched cells were stained with anti-Sca-1 antibodies ( Fig. 3c , left panel). As expected, Sca-1 + population, comprising ∼ 10% of the enriched progenitor cells, showed an increase in mitochondrial volume in MTCH2 F/F Vav1-cre + cells as compared with control cells ( Fig. 3c , right panel). Taken together, these results indicate that loss of MTCH2 results in an increase in both mitochondrial OXPHOS and mitochondrial size/volume. 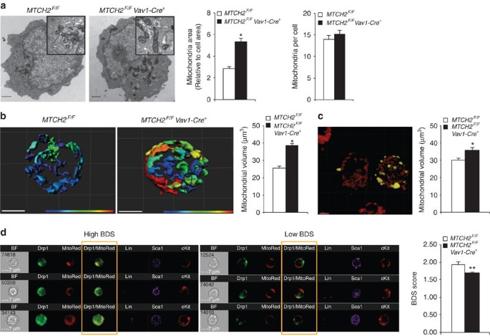Figure 3: Loss of MTCH2 increases mitochondrial size/volume and decreases the mitochondrial levels of Drp-1. (a) Mitochondria are significantly enlarged in MTCH2-deficient progenitors. Shown are representative EM images (left panel; 4,800 × magnification, scale bar 1 μm and 23,000 × magnification, Scale bar, 200 nm, respectively), quantification of mitochondria area (middle panel) and mitochondria number (right panel). Results are presented as mean±s.e.m. (Unpairedt-test, *P<0.05,n=3 mice; 54 fields). (b) Mitochondria volume is significantly increased in MTCH2-deficient progenitors. Left and middle panels: A 3D mitochondrial reconstruction ofMTCH2F/FandMTCH2F/FVav1-cre+CD117+enriched progenitor cells. Scale bar, 3 μm, and the volumetric scale bar, 0.12 μm2–3 μm2. Right panel: Morphometric analysis of 3D reconstructed mitochondria stained with Mitotracker Red. Total mitochondrial volumes ofMTCH2F/FandMTCH2F/FVav1-Cre+CD117+enriched cells are shown. Results are presented as means±s.d. (Unpairedt-test *P<0.05,n=3 mice, 70 fields). (c) Increase mitochondrial volume in Sca-1+progenitors. Left panel: a representative picture ofMTCH2F/FVav1-cre+cells stained with Mitotracker Red (red) and anti-Sca-1 antibody (yellow). Scale bar, 5 μm. Right panel: Morphometric analysis of 3D reconstructed mitochondria stained with Mitotracker Red and positive for Sca-1. Total mitochondrial volumes ofMTCH2F/FandMTCH2F/FVav1-Cre+CD117+enriched Sca-1+cells are shown. Results are presented as means±s.d. (Unpairedt-test *P<0.05,n=3 mice, 70 fields). (d) Reduced Drp-1 co-localization to mitochondria in MTCH2-deficient LSK cells. Cells were stained for Drp-1 (green) and Mitotracker Red, gated for Lin−Sca-1+c-Kit+(LSK), and the co-localization score of the Drp-1 to the mitochondria was calculated using the Bright Detail Similarity (BDS) feature. Left and middle panels: shown are three representative LSK cells with high BDS (high Drp-1/MitoRed co-localization/yellow fluorescence/cells marked by an orange rectangle; left panel) and three representative cells with low BDS (low Drp-1/MitoRed co-localization/lack of yellow fluorescence/cells marked by an orange rectangle; middle panel); scale bar, 7 μm. Right panel: A significantly lower Drp-1/MitoRed co-localization (lower BDS score) was measured for theMTCH2F/FVav1-cre+LSK cells as compared to theMTCH2F/Fcells. Results are presented as mean±s.d. (Unpairedt-test **P<0.01, n=8 mice, 105cells). Figure 3: Loss of MTCH2 increases mitochondrial size/volume and decreases the mitochondrial levels of Drp-1. ( a ) Mitochondria are significantly enlarged in MTCH2-deficient progenitors. Shown are representative EM images (left panel; 4,800 × magnification, scale bar 1 μm and 23,000 × magnification, Scale bar, 200 nm, respectively), quantification of mitochondria area (middle panel) and mitochondria number (right panel). Results are presented as mean±s.e.m. (Unpaired t -test, *P< 0.05 , n =3 mice; 54 fields). ( b ) Mitochondria volume is significantly increased in MTCH2-deficient progenitors. Left and middle panels: A 3D mitochondrial reconstruction of MTCH2 F/F and MTCH2 F/F Vav1-cre + CD117 + enriched progenitor cells. Scale bar, 3 μm, and the volumetric scale bar, 0.12 μm 2 –3 μm 2 . Right panel: Morphometric analysis of 3D reconstructed mitochondria stained with Mitotracker Red. Total mitochondrial volumes of MTCH2 F/F and MTCH2 F/F Vav1-Cre + CD117 + enriched cells are shown. Results are presented as means±s.d. (Unpaired t -test * P < 0.05 , n =3 mice, 70 fields). ( c ) Increase mitochondrial volume in Sca-1 + progenitors. Left panel: a representative picture of MTCH2 F/F Vav1-cre + cells stained with Mitotracker Red (red) and anti-Sca-1 antibody (yellow). Scale bar, 5 μm. Right panel: Morphometric analysis of 3D reconstructed mitochondria stained with Mitotracker Red and positive for Sca-1. Total mitochondrial volumes of MTCH2 F/F and MTCH2 F/F Vav1-Cre + CD117 + enriched Sca-1 + cells are shown. Results are presented as means±s.d. (Unpaired t -test * P < 0.05 , n =3 mice, 70 fields). ( d ) Reduced Drp-1 co-localization to mitochondria in MTCH2-deficient LSK cells. Cells were stained for Drp-1 (green) and Mitotracker Red, gated for Lin − Sca-1 + c-Kit + (LSK), and the co-localization score of the Drp-1 to the mitochondria was calculated using the Bright Detail Similarity (BDS) feature. Left and middle panels: shown are three representative LSK cells with high BDS (high Drp-1/MitoRed co-localization/yellow fluorescence/cells marked by an orange rectangle; left panel) and three representative cells with low BDS (low Drp-1/MitoRed co-localization/lack of yellow fluorescence/cells marked by an orange rectangle; middle panel); scale bar, 7 μm. Right panel: A significantly lower Drp-1/MitoRed co-localization (lower BDS score) was measured for the MTCH2 F/F Vav1-cre + LSK cells as compared to the MTCH2 F/F cells. Results are presented as mean±s.d. (Unpaired t -test ** P<0.01, n =8 mice, 10 5 cells). Full size image Aberrations in the mitochondria fusion/fission machinery [24] , can lead to an increase in mitochondria size and function. Indeed, it was recently demonstrated that improved mitochondrial function correlates with physiological enlargement of mitochondria [25] . Moreover, this mitochondria enlargement was due to less translocation to the mitochondria of the fission protein Drp-1 (ref. 25 ), which is an essential step in fission of the organelle [26] . Thus we assessed the levels of mitochondrial Drp-1 in MTCH2 F/F and MTCH2 F/F Vav1-cre + HSPCs using Imaging Flow Cytometry. Bone marrow cells were stained for Drp-1 (green) and MitoRed, gated for LSK, and the co-localization score of the Drp-1 to the mitochondria was calculated using the Bright Detail Similarity (BDS) feature ( Fig. 3d , left and middle panels; high BDS represents high Drp-1/MitoRed co-localization, yellow fluorescence, and low BDS represents low Drp-1/MitoRed co-localization, lack of yellow fluorescence). Utilizing Unpaired t -test, a significantly lower Drp-1/MitoRed co-localization (lower BDS score) was estimated in the MTCH2 F/F Vav1-cre + cells as compared to the MTCH2 F/F controls ( Fig. 3d , right panel). Thus, MTCH2-deficient cells show less mitochondrial localization of the fission protein Drp-1, suggesting that the increase in mitochondria size and possibly function is due to mitochondrial hyperfusion. However, the precise role of MTCH2 in regulating the translocation of Drp-1 to the mitochondria still remains to be determined. G-CSF mobilization increases mitochondrial OXPHOS and volume To test whether the increase in these mitochondrial parameters is physiologically relevant we analysed these parameters following HSC mobilization and entry into active cell cycle [27] . Mice were injected with granulocyte colony stimulating factor (G-CSF), the most commonly used mobilizing agent for stem cell transplantation [28] , and mitochondrial respiration and mitochondrial size/volume were determined. We found that G-CSF administration led to an increase in both basal and maximal oxygen consumption in enriched progenitors ( Fig. 4a ), and to an increase in mitochondrial volume ( Fig. 4b ), similar to the phenotypes observed in MTCH2 F/F Vav1-cre + cells ( Figs 2 and 3 ). Thus, an increase in mitochondrial OXPHOS and mitochondrial size/volume is associated with HSC mobilization and entry into active cell cycle. 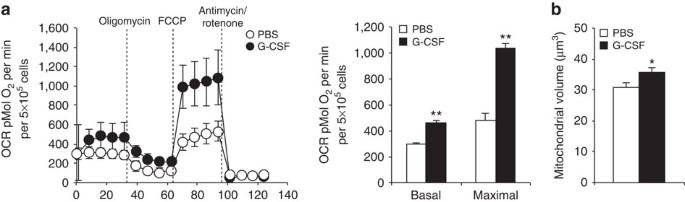Figure 4: G-CSF mobilization increases mitochondrial respiration and volume. (a) Increased mitochondrial respiration upon G-CSF mobilization. Oxygen consumption rates (OCR) were measured in CD117+enriched progenitors using the Seahorse XF24 analyzer. Basal OCR and Maximal OCR (average of results shown in left panel) are shown on the right panel. A representative experiment of three is shown. Results are presented as mean±s.d. (Unpairedt-test, **P≤0.005,n=6). (b) G-CSF mobilization increases the volume of mitochondria. Morphometric analysis of 3D reconstructed mitochondria stained with Mitotracker Red of CD117+enriched progenitor cells following G-CSF mobilization. Total mitochondrial volumes of CD117+enriched progenitors prepared from wild-type mice, either injected with PBS or injected with G-CSF, are shown. Results are presented as mean±s.d. (Unpairedt-test, *P<0.05,n=3 mice, 45 fields). Figure 4: G-CSF mobilization increases mitochondrial respiration and volume. ( a ) Increased mitochondrial respiration upon G-CSF mobilization. Oxygen consumption rates (OCR) were measured in CD117 + enriched progenitors using the Seahorse XF24 analyzer. Basal OCR and Maximal OCR (average of results shown in left panel) are shown on the right panel. A representative experiment of three is shown. Results are presented as mean±s.d. (Unpaired t -test, ** P≤ 0.005, n =6). ( b ) G-CSF mobilization increases the volume of mitochondria. Morphometric analysis of 3D reconstructed mitochondria stained with Mitotracker Red of CD117 + enriched progenitor cells following G-CSF mobilization. Total mitochondrial volumes of CD117 + enriched progenitors prepared from wild-type mice, either injected with PBS or injected with G-CSF, are shown. Results are presented as mean±s.d. (Unpaired t -test, * P < 0.05 , n =3 mice, 45 fields). Full size image Loss of BID phosphorylation primes mitochondrial OXPHOS We next assessed the involvement of BID, the upstream regulator of MTCH2 (ref. 16 ), in regulating mitochondrial function. We previously demonstrated that loss of BID phosphorylation ( BID AA mice), which results in an increase in mitochondrial BID, leads to HSC exit from quiescence [14] . Since both mouse models, BID AA and MTCH2 F/F Vav1-cre + , show loss of HSC quiescence, we suspected that both models would also show similar changes in mitochondrial parameters. Indeed, we found an increase in both basal and maximal oxygen consumption in BID AA enriched progenitor cells ( Fig. 5a ). The increased respiration was accompanied by decreased NADH redox (due to accelerated electron consumption; Fig. 5b ), and an increase in ΔΨm ( Fig. 5c ), similar to the phenotypes observed in the MTCH2 F/F Vav1-cre + cells ( Fig. 2 ). Moreover, electron microscopy analyses of the BID AA progenitors demonstrated a significant increase in mitochondrial size ( Fig. 5d ). Thus, an ‘activating’ mutation in BID and loss of MTCH2 lead to similar phenotypes, arguing that BID acts as a MTCH2 antagonist. 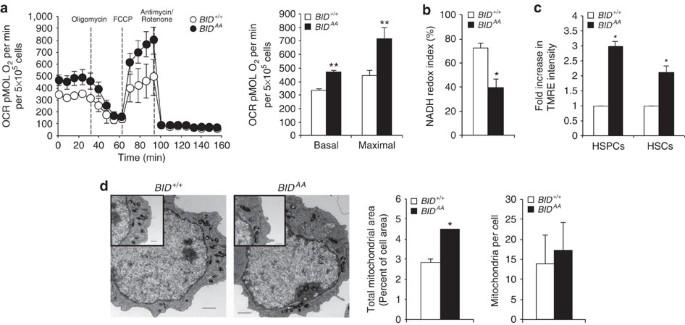Figure 5: Loss of BID phosphorylation primes mitochondrial OXPHOS. (a) Increased mitochondrial respiration inBIDAAenriched progenitors. Oxygen consumption rates (OCR) were measured in CD117+enriched progenitors using the Seahorse XF24 analyzer. Basal OCR and Maximal OCR (average of results shown in left panel) are shown on the right panel. A representative experiment of three is shown. Results are presented as mean±s.d. (Unpairedt-test, **P≤0.005,n=6). (b) Reduced NADH redox inBIDAAHSPCs. NADH redox index was calculated as described in the Methods. Results are presented as mean per cent±s.d. (Unpairedt-test, *P≤0.05,n=4). (c) Increased mitochondrial membrane potential inBIDAAHSCs and HSPCs. Results are presented as mean±s.d. (Unpairedt-test, *P≤0.05,n=4). (d) Mitochondria are significantly enlarged inBIDAAenriched progenitors. Shown are representative EM images (left panel; 4,800 × magnification, scale bar 1 μm and 23,000 × magnification, scale bar, 500 nm, respectively), quantification of mitochondria area (middle panel) and mitochondria number (right panel). Results are represented as mean±s.e.m. (Unpairedt-test, *P<0.05,n=3 mice, 30 fields). Figure 5: Loss of BID phosphorylation primes mitochondrial OXPHOS. ( a ) Increased mitochondrial respiration in BID AA enriched progenitors. Oxygen consumption rates (OCR) were measured in CD117 + enriched progenitors using the Seahorse XF24 analyzer. Basal OCR and Maximal OCR (average of results shown in left panel) are shown on the right panel. A representative experiment of three is shown. Results are presented as mean±s.d. (Unpaired t -test, ** P≤ 0.005, n =6). ( b ) Reduced NADH redox in BID AA HSPCs. NADH redox index was calculated as described in the Methods. Results are presented as mean per cent±s.d. (Unpaired t -test, * P≤ 0.05, n =4). ( c ) Increased mitochondrial membrane potential in BID AA HSCs and HSPCs. Results are presented as mean±s.d. (Unpaired t -test, * P≤ 0.05, n =4). ( d ) Mitochondria are significantly enlarged in BID AA enriched progenitors. Shown are representative EM images (left panel; 4,800 × magnification, scale bar 1 μm and 23,000 × magnification, scale bar, 500 nm, respectively), quantification of mitochondria area (middle panel) and mitochondria number (right panel). Results are represented as mean±s.e.m. (Unpaired t -test, * P <0.05, n =3 mice, 30 fields). Full size image Loss of MTCH2 protects cells from stress-induced death It is well established that physiological enlargement of mitochondria, which correlates with improved mitochondrial function/ATP production, protects cells from stress-induced apoptosis [25] , [29] , [30] . Since the ATM–BID couple is an important regulator of the DNA-damage response in the bone marrow [12] , [14] , [31] we tested the sensitivity of the MTCH2 F/F Vav1-cre + mice to total body irradiation (TBI). Notably, we found that MTCH2 loss provides protection to HSPCs from irradiation-induced death in vivo ( Fig. 6a ), which was also evident in vitro ( Fig. 6b ). In accordance with these findings, the MTCH2 F/F Vav1-cre + progenitors were resistant to TBI-induced caspase-3 activation/cleavage in vivo ( Fig. 6c , Supplementary Fig. 4 ), and MTCH2 F/F Vav1-cre + HSCs were considerably less sensitive to TBI-induced apoptosis ( Fig. 6d ). 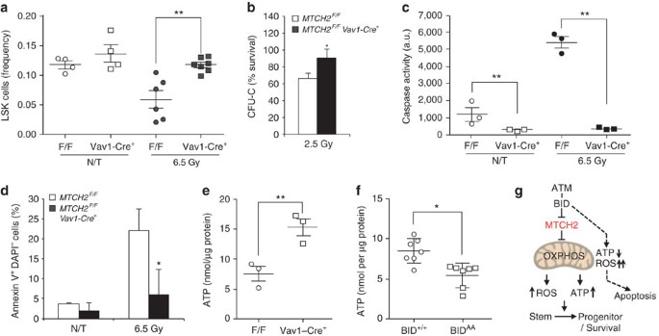Figure 6: Loss of MTCH2 protects cells from stress-induced death. (a) MTCH2-deficient LSK cells are less sensitive to total body irradiation (TBI)-induced death. Mice were subjected to 6.5 Gy TBI, 3 h later were killed and the amount of LSK cells was quantified. Results are presented as mean±s.d. (Unpairedt-test, **P≤0.005,n=4–7). (b) MTCH2-deficient bone marrow cells exhibit unperturbed colony formation in culture following irradiation. Results are presented as mean±s.d. (Unpairedt-test, *P≤0.05,n=3). (c) MTCH2-deficient progenitor cells are resistant to TBI-induced caspase-3 activation. Mice were subjected to TBI, and 30 min later killed and CD117+enriched progenitors were analysed for caspase-3 activity. Results are presented as mean±s.d. (Unpairedt-test, **P<0.005,n=3). (d) MTCH2-deficient HSCs are less sensitive to TBI-induced apoptosis. Mice were subjected to TBI, and a half an hour later killed. Freshly isolated bone marrow was stained for HSC markers (CD150+CD48−CD41−Lin−Sca-1+c-Kit+) together with Annexin V and DAPI for apoptosis detection. Results are presented as means±s.d. (Unpairedt-test, *P<0.05,n=4). (e) Higher basal levels of ATP in MTCH2-deficient progenitors. ATP levels were assessed as described in the Methods. Results are presented as means±s.d. (Unpairedt-test, **P<0.005,n=3). (f) Lower basal levels of ATP inBIDAAprogenitors. ATP levels were assessed as described in the Methods. Results are presented as mean±s.d. (Unpairedt-test, *P<0.05,n=7). (g) Schematic representation of the ATM–BID-MTCH2 pathway regulating mitochondria OXPHOS to determine HSC fate. Figure 6: Loss of MTCH2 protects cells from stress-induced death. ( a ) MTCH2-deficient LSK cells are less sensitive to total body irradiation (TBI)-induced death. Mice were subjected to 6.5 Gy TBI, 3 h later were killed and the amount of LSK cells was quantified. Results are presented as mean±s.d. (Unpaired t -test, ** P≤ 0.005, n =4–7). ( b ) MTCH2-deficient bone marrow cells exhibit unperturbed colony formation in culture following irradiation. Results are presented as mean±s.d. (Unpaired t -test, * P≤ 0.05, n =3). ( c ) MTCH2-deficient progenitor cells are resistant to TBI-induced caspase-3 activation. Mice were subjected to TBI, and 30 min later killed and CD117 + enriched progenitors were analysed for caspase-3 activity. Results are presented as mean±s.d. (Unpaired t -test, ** P< 0.005, n =3). ( d ) MTCH2-deficient HSCs are less sensitive to TBI-induced apoptosis. Mice were subjected to TBI, and a half an hour later killed. Freshly isolated bone marrow was stained for HSC markers (CD150 + CD48 − CD41 − Lin − Sca-1 + c-Kit + ) together with Annexin V and DAPI for apoptosis detection. Results are presented as means±s.d. (Unpaired t -test, * P< 0.05, n =4). ( e ) Higher basal levels of ATP in MTCH2-deficient progenitors. ATP levels were assessed as described in the Methods. Results are presented as means±s.d. (Unpaired t -test, ** P< 0.005, n =3). ( f ) Lower basal levels of ATP in BID AA progenitors. ATP levels were assessed as described in the Methods. Results are presented as mean±s.d. (Unpaired t -test, * P< 0.05, n =7). ( g ) Schematic representation of the ATM–BID-MTCH2 pathway regulating mitochondria OXPHOS to determine HSC fate. Full size image Finally, we assessed the levels of cellular ATP and as expected MTCH2-deficient progenitors possess considerably higher levels of ATP under basal conditions ( Fig. 6e ). Surprisingly, however, we found that the BID AA progenitors possess considerably lower basal levels of ATP ( Fig. 6f ), which seemed consistent with our previous findings that BID AA cells are hypersensitive to irradiation [14] . Interestingly, a recent report [32] argued that an increase in mitochondrial OXPHOS can result in either a significant increase in ATP production, as is the case in the MTCH2 F/F Vav1-cre + cells, or alternatively a significant increase in ROS production (possibly due to a proton leak), as is the case in the BID AA cells since they show a larger increase in ROS ( ∼ 3-fold [14] ) as compared to a ∼ 1.5-fold increase in the MTCH2-deficient cells ( Fig. 2f ). In this study we demonstrate that mitochondrial OXPHOS, regulated by the ATM–BID-MTCH2 pathway, plays a critical role in determining the fate of HSC and progenitor cells ( Fig. 6g ). Our results demonstrate that loss of MTCH2 primes mitochondrial OXPHOS, which acts as a catalyser to drive HSCs into cycle. Since the expression of MTCH2 is considerably higher in restricted progenitor cells (LK cells) as compared with HSPCs (LSK cells), it is possible that MTCH2 suppresses OXPHOS in restricted progenitors and its loss primarily accelerates progenitor differentiation, which, indirectly, drives HSCs into cycle leading to loss of quiescence and finally exhaustion. These results seem opposite from what occurs in T lymphocytes, where resting cells are long lived and possess considerable SRC, whereas when they become activated and start to divide they lose their SRC [33] . Thus, the metabolic requirements for HSC maintenance seem to differ from the metabolic needs of T lymphocytes. The robust increase in mitochondrial OXPHOS in the MTCH2 F/F Vav1-cre + cells correlates with an increase in both basal ATP and basal ROS levels that signal the dormant HSCs to cycle, and concurrently equip them with enough energy to survive increased stress ( Fig. 6g ). On the other hand, the robust increase in mitochondrial OXPHOS in the BID AA cells correlates with a significant increase in basal ROS levels and a decrease in basal ATP levels, which likely contributes to the hypersensitivity of these cells to genotoxic stress ( Fig. 6g ). It should be emphasized that loss of MTCH2 also results in less mitochondrial targeting of BID [16] , which likely contributes to the decreased sensitivity of the MTCH2-deficient cells to genotoxic stress-induced apoptosis. Thus, we identified MTCH2 as a new downstream player in the ATM–BID pathway, at the mitochondria, that via tuning of OXPHOS dictates whether a stem cell will remain quiescent in the bone marrow niche or shift to a migratory cycling and differentiating state replenishing the blood with mature leukocytes. Mice The Weizmann Institute Animal Care and Use Committee approved all animal experiments. MTCH2 F/F mice were generated as described [16] and backcrossed for 10 generations to C57BL6 background. Vav1-Cre male mice (on a C57BL/6 background) were purchased from Jackson Laboratory and bred with MTCH2 F/F females to generate MTCH2 F/F Vav1-Cre + mice. C57BL/6 CD45.1 congenic mice were from the Weizmann Institute of Science and C57BL/6 CD45.2 congenic mice were purchased from Harlan, Rehovot, Israel. BID AA mice were generated as described [14] . TBI experiments were performed as described [14] . All data presented were repeated in at least three independent experiments with 8–10-week-old age and sex-matched mice. Both males and females were used in this study. Respiration Freshly isolated total bone marrow cells were enriched for CD117 + population using Magnetic cell sorting (MACS; Miltenyi Biotec 130-091-224) and 0.5 × 10 6 cells were immobilized to XF 24 plate (Seahorse Bioscience, Cat. # 100777-004) pretreated with Cell-Tak (Corning; Cat#354240). Measurement of intact cellular respiration was performed using the Seahorse XF24 analyzer (Seahorse Bioscience Inc.) and the XF Cell Mito Stress Test Kit according to manufacturer’s instructions and as described [34] . Respiration was measured under basal conditions, and in response to Oligomycin (ATP synthase inhibitor; 0.5 μM) and the electron transport chain accelerator ionophore FCCP (Trifluorocarbonylcyanide Phenylhydrazone; 0.5 μM). FCCP treatment gives two indexes: the Maximal OCR (Oxygen Consumption Rate) capacity of the cells and their spare respiratory capacity (SRC; indicated by maximum OCR calculated as percentage of baseline OCR). Finally, respiration was stopped by adding the electron transport chain inhibitors Rotenone and Antimycin A (1 μM each). NADH Mitochondrial NADH levels were estimated as described [23] . Briefly, mitochondrial NADH was calculated as the difference in arbitrary units between the maximum NADH autofluorescence (in response to 1 mM of potassium cyanide (KCN; Sigma), a potent inhibitor of complex IV resulting in a block in mitochondrial respiration and thus maximum accumulation of mitochondrial NADH); and minimum NADH autofluorescence (in response to 1 μM of the OXPHOS uncoupler FCCP (Seahorse Bioscience Inc.) that induces maximum respiration and thus exhaustion of the mitochondrial NADH pool). NADH redox index was estimated by calculating the initial NADH autofluorescence when the minimum NADH autofluorescence is normalized to 0% and the maximum to 100%. NADH autofluorescence was measured flow cytometrically after excitation with a UV laser with a main emission peak at 470 nm. Transmission electron microscopy Enriched CD117 + progenitor cells were fixed with 3% paraformaldehyde, 2% glutaraldehyde in 0.1 M cacodylate buffer containing 5 mM CaCl 2 (pH 7.4). Than postfixed in 1% osmium tetroxide supplemented with 0.5% potassium hexacyanoferrate tryhidrate and potasssium dichromate in 0.1 M cacodylate (1 h), stained with 2% uranyl acetate in water (1 h), dehydrated in graded ethanol solutions and embedded in Agar 100 epoxy resin (Agar scientific Ltd., Stansted, UK). Ultrathin sections (70–90 nm) were viewed and photographed with a FEI Tecnai SPIRIT (FEI, Eidhoven, Netherlands) transmission electron microscope operated at 120 kV and equipped with an EAGLE CCD Camera. Mitochondria 3D reconstruction and morphometric analysis Enriched CD117 + cells were stained with Pacific Blue anti-Sca1 antibody (1:100 dilution; Biolegend) and mitochondria were stained by incubating the cells for 30 min at 37 °C in IDMEM (Biological Industry, Israel) supplemented with 2% fetal bovine serum (Gibco), 100 nm Mitotracker Red CMXRos (Molecular Probes, Life Technologies). After incubation cells were seeded on Poly- L -Lysine coated slides, fixed for 10 min using fixation solution Cytofix/Cytoperm (BD Biosciences), mounted and visualized on 100 × magnification lens (NA=1.4) using the AX10 Carl Zeiss Microscope with a Yokogawa Spinning Disc (CSU-x1). All the images were taken under the same conditions of laser power and light exposure time. Z-step was set at 0.24 μm and a 3D deconvolution algorithm was applied to the images using Autoquant software (MediaCybernetics). Mitochondrial 3D reconstruction was achieved using segmentation algorithm of Imaris software (Bitplane), and the total mitochondrial volume was calculated for each cell. Flow cytometry For flow cytometric analyses the following monoclonal antibodies were used: c-Kit (105812; clone 2B8), Sca-1 (108116; clone D7), CD150 (115903; clone TC15-12F12.2), CD48 (103409; clone HM48-1), CD41 (13-0411; clone MWReg30), B220 (103204; clone RA3-6B2), CD115 (135506; cloneAFS98), CD11b (101204; clone M1-70), Gr-1 (108406; clone RB6-8C5), Ter119 (116204; clone TER-119), CD3 (100304; clone 145- 2C11) and CD45.1 (110704; clone A20). All the antibodies were purchased from BioLegend, except for antibodies to CD41 (13-0411; clone MWReg30) and B220 (17-0552-81; clone RA3-6B2), which were purchased from eBioscience. All the antibodies were used at a dilution of 1:100. Streptavidin PE/Cy7 (405206) was purchased from BioLegend and used at a dilution of 1:200. All flow cytometric analyses were done using BD LSRII flow cytometer (BD Bioscience). Sorting was done using BD FACSAria cell sorter (BD Bioscience), and data analysis was done using the FlowJo software. Multispectral imaging flow-cytometry (ImageStream) analysis Enriched CD117 + cells were stained with lineage c-Kit, and Sca-1 antibodies (1:100 dilution; Biolegend), and mitochondria were stained by incubating the cells for 30 min at 37 °C with Mitotracker Red CMXRos in HBSS. After incubation cells were fixed in ice for 20 min using fixation solution Cytofix/Cytoperm (BD Biosciences). Next, cells were stained over night with 1:100 mouse anti-Drp-1 antibody (BD Transduction Laboratory; Cat. N.611112); and the following day cells were incubated with FITC conjugated goat anti-mouse (Jackson ImmunoResearch Laboratories) antibody at a concentration of 1:200 for 30 min. Cells were imaged using multispectral imaging flow cytometry (ImageStreamX, Amnis Corp). For multispectral imaging flow cytometry, approximately 10 5 cells were collected from each sample and data were analysed using image analysis software (IDEAS 6.1; Amnis Corp). Images were compensated for fluorescent dye overlap by using single-stain controls. Cells were gated for single cells using the area and aspect ratio features, and for focused cells using the Gradient RMS feature, as previously described [35] . Cells were further gated for Lin – and then gated for Sca-1 + c-Kit + , based on their pixel intensities. The co-localization of Drp-1 with the mitochondria was quantified using the BDS feature (the log transformed Pearson’s correlation coefficient of the localized bright spots in the two input images) [35] . G-CSF Mice were injected i.p. with G-CSF, Filgrastim (Kirin-Amgen Inc.; 90 μg kg −1 in 200 μl of PBS) for three consecutive days (48 h total). Control mice received vehicle only injections. Mice were killed 1 h post last injection. Bone marrow was flushed, enriched and used for the studies described. ATP and lactate measurements CD117 + enriched cells were lysed with Promega cell lysis buffer (E1531) and: (1) ATP levels were measured using the ATPlite Luminescent kit (PerkinElmer) according to the manufacturer’s instructions; (2) Lactate levels were measured using the Lactate kit according to manufacturer’s instructions (Biovision Incorporate, Lactate Assay kit Cat. K607). Cell cycle To analyze quiescence of cells, total bone marrow cells stained for the designated markers were fixed, permeabilized using the Cytofix/Cytoperm kit (BD Bioscience) and stained with the Ki-67 antibody (BD Bioscience) and DAPI (4′,6-Diamidino-2-phenylindole dihydrochloride; 5 μg ml −1 ; Sigma). To determine the proliferation status of cells, mice were given one daily dose of BrdU (5-Bromo-2-DeoxyUridine; 3.3 mg per mouse) by i.p. injections for three consecutive days, and mice were killed for analysis 2 h following the last administration. BrdU incorporation was assessed using the BrdU Flow kit (BD Bioscience), according to the manufacturers’ instructions. Colony-forming assay For colony-formation assays, 100,000 bone marrow mononuclear cells were plated in methyl cellulose (R&D Systems) supplemented with fetal bovine serum, Pen-strep and 10 ng ml −1 of IL-3, IL-6, SCF, GM-CSF, M-CSF, G-CSF (Peprotech). Colony number (CFU-C) was enumerated following 7 days in culture. Competitive bone marrow transplantations Lethally irradiated C57BL/6-CD45.2 mice were transplanted with 2.5 × 10 6 of either MTCH2 F/F or MTCH2 F/F Vav1-Cre + mice (CD45.2) bone marrow mononuclear cells in competition with 2.5 × 10 6 wild-type (CD45.1) competitor bone marrow mononuclear cells (1:1 ratio). Lethally irradiated (9.5 Gy) recipients were given a broad-spectrum antibiotic in drinking water (Cyproxine 200, Bayer) one day before transplantation. Reconstitution of donor-derived cells (CD45.2 + ) in peripheral blood was monitored, once every 2 weeks, by staining with antibodies against CD45.1. Long-term reconstitution of the bone marrow LSK and HSC cells was evaluated at 20 weeks post transplantation by staining total bone marrow cells with CD45.1 and HSC markers. Quantitative real-time PCR RT-PCR was done as previously described [14] . Primer sequences used for all the genes tested are listed below: MTCH2 F- 5′-TGTTCACAGGCTTGACTCCA-3′ MTCH2 R- 5′-CAAACTGTATAGGTGAATGGCTCT-3′ Ndufs8 F- 5′-GACTGGGCATGACCCTAAGTT-3′ Ndufs8 R- 5′-CGCTCCTCTCCAGATGGGTA-3′ SDHb F- 5′-AATTTGCCATTTACCGATGGGA-3′ SDHb R- 5′-AGCATCCAACACCATAGGTCC-3′ Cox5b F- 5′-ACCCTAATCTAGTCCCGTCC-3′ Cox5b R- 5′-CAGCCAAAACCAGATGACAG-3′ ATP5a1 F- 5′-CATTGGTGATGGTATTGCGC-3′ ATP5a1 R- 5′-TCCCAAACACGACAACTCC-3′. ROS ROS levels (superoxide anion) were assessed by 20 min incubation at 37 °C of bone marrow cells with 5 μM hydroethidine (DHE; Molecular Probes, Life Technologies) for cellular ROS or 10 μM MitoSOX (Molecular Probes, Life Technologies) for mitochondrial ROS. Cells were then washed once with PBS and stained for HSC markers. Fluorescence of oxidized DHE or MitoSOX was determined flow cytometrically. Mitochondrial membrane potential Total bone marrow cells were incubated with 50 nm Tetramethylrhodamine ethyl ester perchlorate (TMRE; Enzo Life Sciences) for 20 min at 37 °C, washed once with PBS and stained for HSC markers. Fluorescence of TMRE was determined flow cytometrically. For mitochondrial mass estimation, 100 nm Mito Tracker Green (MTG; Molecular Probes) was added together with TMRE. Annexin V staining Mice were either left untreated or subjected to TBI and 0.5 h later mice were killed. Freshly isolated bone marrow was stained for flow cytometric analysis. Annexin V detection kit (BD Biosciences) was used according to manufacturer’s instructions, coupled with DAPI (Sigma) staining for dead cells. Caspase-3 activity Mice were either left untreated or subjected to TBI and 0.5 h later total bone marrow cells were enriched for CD117 + population using Magnetic cell sorting (MACS; Miltenyi Biotec 130-091-224). Enriched cells were lysed with Promega cell lysis buffer (E1531) and caspase activity was estimated using Caspase-Glo 3/7 Luminescent Assay kit (Promega) according to manufacturer’s instructions. Western blot Western blot analysis was performed as previously described [16] . Antibodies used for western blotting included anti-cleaved caspase-3 (Cleaved Caspase-3 (Asp175) Antibody 9661s; 1:1,000 dilution; Cell Signaling) and anti-βActin (A1978; 1:5,000 dilution; Sigma). Statistical analysis P -values were calculated by using an unpaired Student’s t -test. How to cite this article: Maryanovich, M. et al . An MTCH2 pathway repressing mitochondria metabolism regulates haematopoietic stem cell fate. Nat. Commun. 6:7901 doi: 10.1038/ncomms8901 (2015).